Larger mammals have longer faces because of size-related constraints on skull form Facial length is one of the best known examples of heterochrony. Changes in the timing of facial growth have been invoked as a mechanism for the origin of our short human face from our long-faced extinct relatives. Such heterochronic changes arguably permit great evolutionary flexibility, allowing the mammalian face to be remodelled simply by modifying postnatal growth. Here we present new data that show that this mechanism is significantly constrained by adult size. Small mammals are more brachycephalic (short faced) than large ones, despite the putative independence between adult size and facial length. This pattern holds across four phenotypic lineages: antelopes, fruit bats, tree squirrels and mongooses. Despite the apparent flexibility of facial heterochrony, growth of the face is linked to absolute size and introduces what seems to be a loose but clade-wide mammalian constraint on head shape. Mammals range in size from minute shrews to gigantic whales [1] . The morphological disparity in their cranial shape is extraordinary, as every visitor to a natural history museum appreciates. Despite the scale of differences between major, and even minor, clades, the covariance structure in the mammalian skull seems to be highly conserved [2] , [3] , [4] , [5] . How the profound variety of skull forms was generated from such a seemingly conservative system is a fundamental and largely open evolutionary question. Correlated variation, known as allometry when it results in proportional changes relative to size, may facilitate the rapid origin of differences among closely related species [2] , [4] , [6] . Allometry is known to be a major component of covariation in the mammalian cranium [7] and contributes to its integration and modularity [8] . Indeed, without integration, fundamental functions could be compromised as size changes during ontogeny and in evolution [9] , [10] . Integration probably explains why the proportional length and orientation of the cranial base and face account for a large amount of variation in dogs and humans [11] . Consequently, small differences in the genetic regulation of growth factors can, by altering size, indirectly but readily affect shape. Allometry thus acts in evolution both as a constraint by reducing the range of directions of shape change, and as an accelerator by producing pronounced phenotypic differences along lines of least evolutionary resistance [12] , [13] . For instance, in papionins, mandrils and baboons the evolution of bigger sizes and longer faces has followed similar, although non-identical, allometric trajectories, as members of each clade became less arboreal and incorporated a wider variety of foods in their diet compared with their closest relatives, the hard-fruit-eating and short-faced mangabeys [14] . Craniofacial elongation is a common aspect of postnatal growth in mammals. Human babies, as well as most, if not all, other juvenile placental mammals, have small faces relative to big and comparatively round heads. The face subsequently grows faster than the braincase, making the head less globular and the jaws more prominent. The evidence of a size-related trend from brachycephaly to dolichocephaly in the ontogeny raises intriguing questions about a similar trend in macroevolution: is there a general species-level correlation between size and dolichocephaly? Might the correlation actually be a common occurrence among closely related species across a wide range of placental orders? To investigate the answers to these questions, we assessed size-related craniofacial changes using statistical shape analysis on three-dimensional (3D) anatomical landmarks in four speciose, ecomorphologically and phylogenetically disparate groups of placental mammals: antelopes (Cetarctiodactyla: Antilopinae and Cephalophinae); fruit bats (Chiroptera: Pteropodinae); African mongooses (Carnivora: Herpestinae); African tree squirrels (Rodentia: Sciurinae). These four lineages all originated in the Miocene (~15–25 million years ago) and have their most recent common ancestor in the deepest part of the Eutherian tree [15] , [16] , [17] . The groups have a range of cranial sizes more than twofold within the groups and tenfold among them. The study confirms that a pervasive effect of size-related craniofacial shape variation, strongly reminiscent of that found within species during ontogeny, occurs across adults of closely related species of placentals. Larger animals are generally long-faced and small ones have proportionally larger braincases. That the pattern is broadly similar across four orders of mammals, whose divergence started soon after (if not before) the extinction of dinosaurs, suggests that it might be a ‘rule’ with few exceptions in the adaptive radiations of placentals. 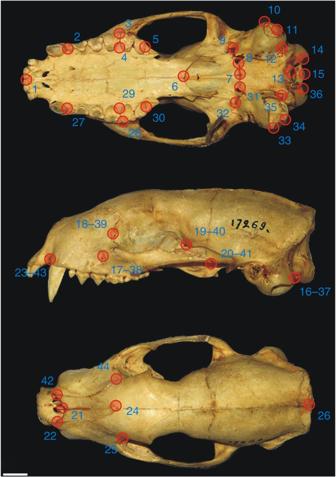Figure 1: Landmark configuration. In side view, the number for the corresponding matching landmark on the right side is shown next to the left side landmark. Scale bar=1 cm. 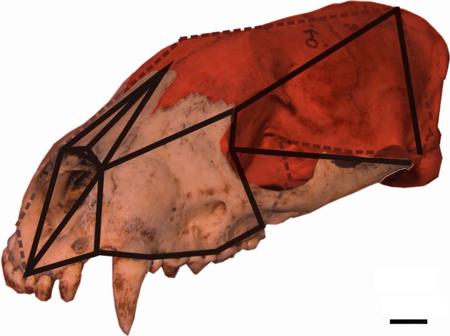Figure 2: Wireframe. Links between landmarks used inFigs 3and4to aid the visualization of shape variation. Dotted lines are used for linking landmarks on the right side, which is not visible. Links for cranial base and occipital landmarks are not shown to simplify the diagram. Light and dark red colours emphasize the face and the braincase, respectively. Scale bar=1 cm. Size-related shape trends The four lineages (cranial landmarks shown in Figs 1 and 2 and defined in Table 1 ; samples described in Table 2 ) occupy distinct, parallel regions of the first three axes of form space (96.1, 1.7 and 1.0% of total variance, respectively) ( Fig. 3 ). PC1, the vector dominated by size and representing the shared allometric variation in shape, defines the main trajectory of each group. 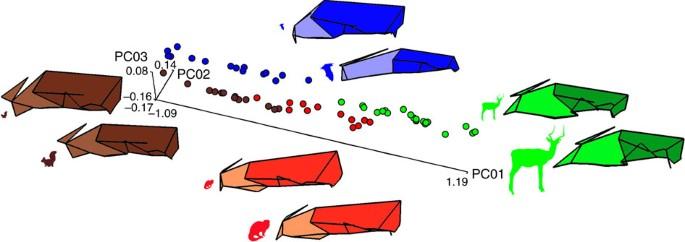Figure 3: Procrustes form space trajectories. The colour code for symbols, shape diagrams and icons is green for antelopes, blue for bats, red for mongooses and brown for squirrels. Icons are roughly proportional to opposite extremes of cranial size within each group. Wireframe shape diagrams, with the face emphasized using lighter colours, help to visualize 3D cranial landmark configurations (in side view) at of the group-specific form trajectories. The allometric relationship was significant in all four groups and explained 10–50% of the variances ( Table 3 ). The regression trajectories (summarized in Fig. 4 ) were less divergent between groups than expected by chance. Each of the four trajectories showed that larger species have proportionally longer faces (light-coloured region, Figs 3 and 4 and Supplementary Movies 1–4 ) relative to the braincase (dark-coloured region). The parallel is particularly pronounced in antelopes and bats. Some aspects of allometric variation are lineage-specific. For instance, in squirrels cranial flexion and brachycephaly are both found in smaller species. Figure 1: Landmark configuration. In side view, the number for the corresponding matching landmark on the right side is shown next to the left side landmark. Scale bar=1 cm. Full size image Figure 2: Wireframe. Links between landmarks used in Figs 3 and 4 to aid the visualization of shape variation. Dotted lines are used for linking landmarks on the right side, which is not visible. Links for cranial base and occipital landmarks are not shown to simplify the diagram. Light and dark red colours emphasize the face and the braincase, respectively. Scale bar=1 cm. Full size image Table 1 Landmark description. Full size table Table 2 Samples *: A, antelopes; B, bats; M, mongooses; S, squirrels. Full size table Figure 3: Procrustes form space trajectories. The colour code for symbols, shape diagrams and icons is green for antelopes, blue for bats, red for mongooses and brown for squirrels. Icons are roughly proportional to opposite extremes of cranial size within each group. Wireframe shape diagrams, with the face emphasized using lighter colours, help to visualize 3D cranial landmark configurations (in side view) at of the group-specific form trajectories. Full size image Table 3 Allometric trajectories. 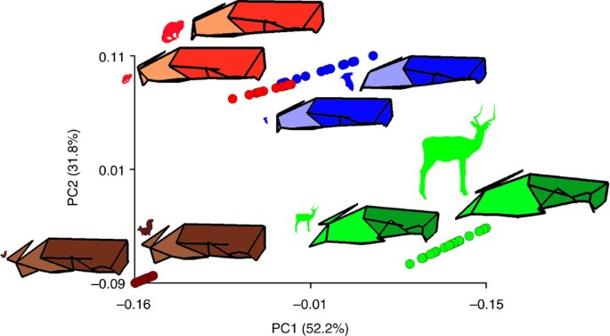Figure 4: Regression trajectories. Lineage-specific allometric trajectories summarized using a principal component analysis of group-specific predictions. Trajectories accounting for 84% of total allometric variance are clearly pointing to similar directions. Wireframe shape diagrams, with the face emphasized using lighter colours, help to visualize 3D cranial landmark configurations (in side view) at opposite extremes opposite extremes of the trajectories of each group. Full size table Figure 4: Regression trajectories. Lineage-specific allometric trajectories summarized using a principal component analysis of group-specific predictions. Trajectories accounting for 84% of total allometric variance are clearly pointing to similar directions. Wireframe shape diagrams, with the face emphasized using lighter colours, help to visualize 3D cranial landmark configurations (in side view) at opposite extremes opposite extremes of the trajectories of each group. Full size image Conserved pattern The mean angle between the allometric vectors of the four groups (72.9°) was smaller than expected by chance ( P =0.017 for males, P =0.03 for females) and 16 out of 24 pairwise tests (females, males, without or with comparative methods— Table 3 ) were highly significant even after Bonferroni correction for 24 simultaneous tests (Permutation test: P <0.0004). Not all size-related variation in cranial shape was linked to the proportional length of the face. This is why angles between some of the allometric vectors were comparatively wide, as expected in clades whose dental and cranial structures are as diverse as these. However, a strong allometric component was clearly related to facial length, as indicated by both the P -values ( Table 3 ) and inspection of the allometric shape models ( Figs 3 and 4 and Supplementary Movies 1–4 ). Note that a vector angle of 0° indicates exact parallelism, an angle of 90° indicates zero parallelism, and one of 180 indicates perfect reverse parallelism. Although the mean angle between our allometric vectors is closer to 90 than to 0°, it is significantly smaller than expected by change because of the shared allometry in facial length. As our tests show, an angle as small as 72.9° in a 60-dimensional-shape space has a vanishingly small probability of occurring by chance. Further, as the diagrams illustrate, the non-parallel allometric component is related to clade-specific differences in the overall skull shape, whereas the parallel allometric component (dominant in Figs 3 and 4 ) corresponds to facial length relative to size. It is this shared component that contributes to statistical significance in the test for parallel trajectories. Thus, despite their clade-specific phenotypic and ecological differences, all these four groups share a clear common pattern: bigger species are dolichocephalic and their smaller relatives are brachycephalic. The similarity of allometric trajectories indicate that facial length scales not only with ontogenetic growth [18] , but is an evolutionary allometry associated with adult size that is conserved among clades that diverged soon after or even before the dinosaur extinction (that is, ca. 65 mya). A large component of the facial variation in mammals may, therefore, be associated with their diversity of size, which is orders of magnitude greater than in other vertebrate groups. The covariation between the face and braincase operates both as a constraint, channelling variation along predictable lines, and as a source of variation related to differences in diet and appearance [19] . The constraint is implied by the tight linear axes in the form space. Evolution along those axes allows disparate shapes to arise more quickly than if evolutionary pathways followed a diffusive random walk through the morphospace. Facial shape itself can therefore respond to selection by a simple change in body size [13] , as in South American monkeys in whom a large range of craniofacial differences have arisen along with variation in size as a response to dietary specialization [20] . Shortening of the face is characteristic of domestication in mammals, which often selects for smaller size, and has been reported in pigs, cattle, dogs and cats [21] . In mice mutants, relatively small brains co-occur with prognathic faces [19] , [22] . This covariation among anatomical parts can result from gene pleiotropy and linkage, from developmental interactions between pathways or tissues, from the cross-tissue action of hormones or the epigenetic action of muscles or environmental factors on bones [22] , [23] , [24] . Emerson and Bramble [9] , who discussed the possibility of negative allometry between the cerebral skull and face in carnivores and ungulates, suggested a biomechanical explanation that might contribute to the pattern we observe. To maintain isometry relative to body mass, the brain should scale with exponent 1 and the length of the jaw with exponent 1/3. When the jaw length is related to brain size (and therefore braincase size), an increase in body mass would generate a relatively smaller jaw with potentially negative biomechanical or adaptive consequences (smaller feeding apparatus in relation to the brain and proportionally less space in the head for powerful masticatory muscles in larger animals). In fact, however, the brain generally scales with a 3/4 exponent relative to body mass [25] , which is similar to a most common, although non-universal, exponent for the scaling of metabolism [26] . Then, if the brain grows less and the jaw more rapidly relative to body mass, one might expect a degree of negative and positive allometry in the braincase and in the jaw, respectively. The possible role of heterochrony in phenotypic evolution has stimulated scientific discussion, especially in the context of human evolution. A neotenic hypothesis of human origin, although inspiring, is controversial and unlikely to hold in a narrow-sense [27] . Regardless of the fine details, the shortening of the face in such a large animal, as us humans, is an exception to the allometry between size and facial proportions that generally holds for mammals. One of the proximate reasons why our face is unusually short for our body size is that we need to accommodate a large, rapidly growing brain that forces the facial prominences to be spread apart as they begin to elongate [22] . The enlargement of the brain, the progressive reduction in canines and molars and an increasing reliance on preprocessed food, which reduces the need of powerful masticatory muscles, may have overcome in our lineage the basic allometric facial constraint that we have identified, allowing humans to evolve an unusual phenotype in terms of cranial proportions. If the shared size-related allometry of facial proportion holds in primates (as, for instance, had been suggested at a macroevolutionary level in several groups of Old World monkeys [14] , [28] , [29] ), and acts as an evolutionary shortcut to facilitate the production of phenotypic variation in the transition from micro- to macro-evolution, exceptions to the 'rule' will provide key evidence to our understanding of the origin of deep morphological and ecological divergence in the hominins as well as in other lineages. Specimens Adult specimens from the collection of the Royal Museum for Central Africa (Tervuren, Belgium) and the La Specola Natural History Museum (Florence, Italy) were selected based on dentition and complete closure of sutures. Crania were measured using a Microscribe 3D digitizer. Three-dimensional Cartesian coordinates of anatomical landmarks were recorded on one side (the left one) to reduce digitization time and thus increase the number of specimens measured during the time available for data collection. The loss of information implied by this approach is minimal especially in the context of macroevolutionary studies, which do not investigate asymmetry. Asymmetry, if present is unlikely to account for more than a tiny fraction of the total variance, as suggested by a visual inspection of specimens and the absence in the literature of any reference to an evident asymmetry in the study groups. To improve the effectiveness of the visualization and the accuracy of the superimposition, however, symmetric landmarks were mirror reflected and the tiny asymmetric component of landmarks on the midplane was removed [30] . The mirror reflected landmark configuration is shown in Fig. 1 and the description of the landmark configuration is presented in Table 1 . The wireframe diagram [31] used to aid the visualization of shape variation is shown in Fig. 2 . A list of taxa and sample sizes is available in Table 2 . Overall, more than 700 individuals from 61 species described using 44 3D cranial landmarks were analysed. Analyses were performed using separate samples for females and males in antelopes and bats because they generally are sexually dimorphic. However, results were virtually identical in the two sexes and are therefore shown in these two lineages using males only. Measurement error was tested on a subsample of specimens, each repositioned and redigitized twice, using a hierarchical analysis of variance [31] , [32] to control for the effect of lineage, species and sex. Individual variation in size and shape was significantly larger than differences between replicas (MANOVA: size: F 3,41 =12,393.63, P <0.0001; shape: F 213,2911 =18.75, P <0.0001). Geometric morphometric and statistical analysis Differences in the position of the specimens during the process of data collection were removed and size separated from shape using a generalized Procrustes analysis [33] . Size was estimated using centroid size, the square root of the sum of squared distances of each landmark from the centroid of the configuration. Centroid size was highly correlated ( R =0.983) to cranial length, which is a common proxy for body size [34] . For this reason, and for the sake of brevity, here and in most other sections, we referred to cranial centroid size simply as size. Size and shape were averaged within species. Size was transformed using the natural logarithm and appended to the matrix of Procrustes shape coordinates to perform a principal component analysis (PCA) in the Procrustes form space [35] , [36] , [37] . PC1 is therefore dominated by size and summarises the pooled within group allometry, which represents the ‘common allometric component’ (p. 684) (ref. 36 ). Scatterplots of the first PCs in the Procrustes form space can be used to quantitatively describe the main aspects of morphological change and explore differences and similarities across groups. In this morphospace, the four groups have strong parallels in skull shape, despite their profound clade-specific differences. However, the appearance of parallel trends can arise as an artifact of form space because size and shape are measured in different units, and the form space is just a simple and effective way of summarizing in a single scatterplot both size and allometric variation. To avoid this pitfall in Fig. 3 , we modelled the shapes of each clade in lineage-specific form spaces at their large and small extremes using wireframe diagrams and qualitatively assessed where the trend was dominated by facial elongation. For the same reasons, we did not test vectors between PCs in the form space but did test for facial allometry within each lineage by regressing multivariate shape onto the natural logarithm of size and in Fig. 4 summarized the corresponding trajectories with a principal component analysis of allometric shapes predicted by lineage-specific regressions [38] . Tests were performed on the raw data first and then again taking phylogenetic relatedness into account based on the supertree of Bininda-Emonds et al . [39] Significance was assessed using a 10,000 permutation test for the proportion of variance explained by the independent variable (that is, log-size) Finally, we tested whether the relationship between size and facial shape was less divergent than expected by chance using a vector randomization method [40] . Thus, angles between pairs of allometric vectors estimated by the regressions within groups were computed as inner dot products. Then, to determine whether observed angles were significantly smaller (more parallel) than expected by chance, they were tested relative to the distribution of simulated randomized vectors obtained using 10,000 permutations of the size variable [40] , [41] , [42] . As for the regressions, all tests of angles were performed using both the original variables and phylogenetic independent contrasts (PIC) [43] , which take the non-independence of observations due to phylogeny [39] into account. With 44 3D landmarks and 61 species means, there are 60 dimensions in which these taxa can vary in the Kendall shape space and angles can range from 0 to 180. That and the fact that the four clades are extremely different in facial shape and specialization means that we do not expect an exact parallelism between size and shape in all 60 shape variables. However, if our hypothesis about facial constraint is correct and the allometric pattern is strong within each group, we do expect the divergence to be significantly smaller than expected by chance and that the aspects of shape that are related to size will largely involve the proportional length of the face. Analyses were performed in the following programs [42] , [44] , [45] , [46] , [47] : MorphoJ, Morpheus et al ., Morphologika, NTSYSpc and Mathematica. How to cite this article: Cardini, A. et al . Larger mammals have longer faces because of size-related constraints on skull form. Nat. Commun. 4:2458 doi: 10.1038/ncomms3458 (2013).